Ultra-rapid access to words in the brain Rapid information processing in the human brain is vital to survival in a highly dynamic environment. The key tool humans use to exchange information is spoken language, but the exact speed of the neuronal mechanisms underpinning speech comprehension is still unknown. Here we investigate the time course of neuro-lexical processing by analyzing neuromagnetic brain activity elicited in response to psycholinguistically and acoustically matched groups of words and pseudowords. We show an ultra-early dissociation in cortical activation elicited by these stimulus types, emerging ∼ 50 ms after acoustic information required for word identification first becomes available. This dissociation is the earliest brain signature of lexical processing of words so far reported, and may help explain the evolutionary advantage of human spoken language. The human brain has evolved to support rapid information processing, enabling us to react appropriately and in a timely manner to events in the constantly changing world around us, a skill vital to our biological survival. Our key communication tool, speech, is a stream of rapidly changing complex sounds. During linguistic processing, acoustic information contained in speech signals is passed from the cochlea to the neocortex extremely quickly, in ∼ 15–20 ms [1] , [2] , and it takes just ∼ 10–30 ms for neural information transfer from superior-temporal core-auditory and linguistic areas to the inferior-frontal cortex, which is also involved in speech and language processing [3] , [4] , [5] . A network of key regions for language processing may therefore ignite within 50 ms of the information arriving at the ear, providing a neurobiological basis for rapid linguistic processing, word recognition and comprehension. A key component of linguistic processing is lexical access and selection—the mapping of sounds onto representations in the mental lexicon. Influential psycholinguistic accounts of spoken word recognition have long emphasized the speed of lexical processing [6] , [7] , [8] , but, to date, neurobiological correlates of the psycholinguistic processes at such early times are unknown. To track the dynamic nature of lexical processing, temporally resolved neurophysiological imaging tools such as electroencephalography (EEG) and magnetoencephalography (MEG) are ideal because they make it possible to measure the corresponding brain activity non-invasively with millisecond time resolution. To date, most studies using such neurophysiological methods have been in the visual domain and have reported neural correlates of lexical processing peaking at 350–400 ms after presentation of written words [9] , [10] , [11] , [12] , with some studies arguing that lexical processes start within 200 ms after display onset [13] , [14] , [15] , [16] . Similar post-onset latencies were reported in the auditory domain [17] , [18] , [19] , where the majority of previous studies focussed on top-down lexical effects driven by wider sentence contexts rather than single word access per se . Importantly, unlike written words, which are displayed whole, spoken words unfold over time and therefore average measurements made relative to the onsets of various words whose recognition points vary, are difficult to interpret in terms of the neural dynamics of word recognition processes. Therefore, experimental work in the auditory domain, the native modality of human language, requires precise knowledge of the critical point in time when words can first be recognized based on the temporally evolving acoustic speech signal [20] . Previous research investigating the lexical processing of single spoken words using strictly matched word and pseudoword stimuli, proposed the earliest neural correlates of access to lexical representations at 100–200 ms after presentation of acoustic information allowing the stimulus to be identified (for review, see ref. 21 ). This is still later than the speed that would be possible in theory; furthermore, studies reporting lexicality effects at such early latencies using auditory stimuli have usually relied on an unnaturally high rate of repetition of just a few stimuli in the so-called mismatch negativity (MMN) paradigm [22] . Thus, the speed of neural access to spoken word information has remained controversial and the putative early neural correlates of lexical processing have not been documented until now. Here we show differences in the amplitude of MEG brain responses to words and pseudowords emerging as early as 50 ms after the presentation of acoustic information required for word recognition. The effect, which appears to be underpinned by perisylvian cortical structures, may reflect the earliest stages of lexical access. We investigated the time course of lexical processing of spoken words by comparing listeners' ( n =22) neuromagnetic brain responses to 108 distinct meaningful words (consonant-vowel-consonant (CVC) structure, for example, joke and boat) with a set of 108 word-like and phonotactically legal but meaningless pseudowords (for example, jote and boak) that were matched on a number of psycholinguistic and acoustic properties ( Supplementary Fig. S1 ; for stimulus details see Methods). To tailor stimuli to the needs of neurophysiological imaging, all stimuli ended in an unvoiced plosive. Whereas the onset consonant of each stimulus and the subsequent vowel were associated with a range of lexical representations for both the words and the pseudowords (the so-called 'cohort'), it was the stimulus-final stop consonant that determined lexical status either as a unique English word or as a meaningless pseudoword. A separate psycholinguistic gating study (for methods, see ref. 23 ) performed with all 216 stimuli by participants not taking part in the MEG study investigated the word recognition point for each stimulus, that is, the critical point in time where stimuli could be first identified. Results confirmed that the words were recognized at the onset of the syllable-final stop consonant. Previous neurophysiological and neurocomputational research showed that the neurophysiological difference between word and pseudoword processing is influenced by attention. As reliably stronger responses to words than pseudowords were found when subjects did not attend to stimuli, and early neurophysiological effects may be masked by focused attention, [24] , [25] participants' attention was diverted from the stimuli in the present experiment; they were instructed to attend to a silent film while listening passively to the auditory stimuli. Their performance on the film-watching task was later assessed through a questionnaire. Neuromagnetic brain activity was recorded from a high-density whole-head MEG set-up (Vectorview, Elekta-Neuromag, Helsinki) and event-related magnetic fields were calculated relative to the word recognition point (final plosive). Sensor-level effects Time windows for analysis were identified from peaks in the global signal-to-noise ratio (SNR) calculated over all stimuli and sensors in the grand average across participants. For statistical analysis, data were first quantified as the absolute magnetic field amplitude of the 102 orthogonal planar gradiometer pairs ( Fig. 1a ). 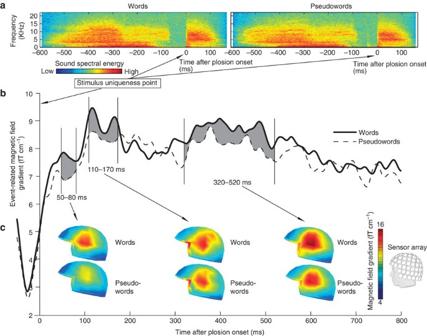Figure 1: MEG sensor-level effects. (a) Spectrogram of the average of all 108 word and all 108 pseudoword sound files created relative to the stimulus uniqueness points. Words and pseudowords were matched on acoustic phonetic as well as psycholinguistic properties, thus differences in the brain responses to the two types of stimuli can only be attributed to lexical status. (b) Global event-related magnetic field gradients observed in response to real words and pseudowords: square root of the sum of squares of the amplitudes of the two gradiometers in each pair averaged over all gradiometer pairs and across all participants (n=22). Data are shown relative to the mean onset of the stimulus uniqueness point (stimulus-final plosion). Three time windows are highlighted corresponding to those selected for statistical analysis based on the peaks of the signal-to-noise function computed over all stimuli and sensors. (c) Topographic field gradient maps (left view) show the distribution of the activations averaged over each of the three time windows, for words and pseudowords separately. Figure 1: MEG sensor-level effects. ( a ) Spectrogram of the average of all 108 word and all 108 pseudoword sound files created relative to the stimulus uniqueness points. Words and pseudowords were matched on acoustic phonetic as well as psycholinguistic properties, thus differences in the brain responses to the two types of stimuli can only be attributed to lexical status. ( b ) Global event-related magnetic field gradients observed in response to real words and pseudowords: square root of the sum of squares of the amplitudes of the two gradiometers in each pair averaged over all gradiometer pairs and across all participants ( n =22). Data are shown relative to the mean onset of the stimulus uniqueness point (stimulus-final plosion). Three time windows are highlighted corresponding to those selected for statistical analysis based on the peaks of the signal-to-noise function computed over all stimuli and sensors. ( c ) Topographic field gradient maps (left view) show the distribution of the activations averaged over each of the three time windows, for words and pseudowords separately. Full size image Significantly enhanced brain responses to real words compared with matched pseudowords were observed in three time windows ( Fig. 1b ). The first difference emerged surprisingly early, already at 50–80 ms, following the word recognition point (7.71 fT cm −1 for words versus 6.94 fT cm −1 for pseudowords, t(21)=1.941, P =0.033). A subsequent lexicality effect, at 110–170 ms, confirmed a pattern known from previous studies investigating the MMN brain responses to spoken words and pseudowords (8.98 versus 8.38 fT cm −1 , t(21)=2.580, P =0.009); in the N400 time window the difference between words and pseudowords was again significant (320–520 ms: 8.69 versus 8.16 fT cm −1 , t(21)=0.049). In all the three time windows, words elicited stronger event-related fields than pseudowords. The effects were maximal and significant at left fronto-temporal sensors ( Fig. 1c ; Supplementary Fig. S2 : 50–80 ms: 9.15 versus 7.85 fT cm −1 , t(21)=2.578, P =0.009; 110–170 ms: 10.26 versus 9.37 fT cm −1 , t(21)=1.970, P =0.031 and 320–520 ms: 10.73 versus 9.80 fT cm −1 , t(21)=2.292, P =0.016). No significant effects were observed over the right hemisphere. No significant effects were seen before the uniqueness point. Cortical sources underlying sensor-level effects Following the sensor-space analysis, neural generators underlying activations registered through all 306 MEG sensors were estimated using distributed current source models (L2 Minimum Norm Estimation ref. 26 ,) restricted to cortical gray matter defined on the basis of individual participant's structural MR images, and morphed to the group average brain for grand averaging ( Fig. 2 ). Statistical analyses focused on source activations in the three time windows identified at the sensor level. Regions of interest (ROIs) were selected for analysis on the basis of the maximal source activations calculated across all stimuli in the grand average across participants ( Supplementary Fig. S3 ). 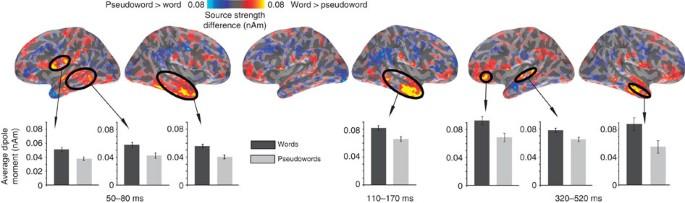Figure 2: Cortical sources underlying MEG sensor-level effects. Differences in minimum-norm source estimation of the brain responses elicited by words and pseudowords, averaged over all participants (n=22). Images show mean source strength averaged across three windows corresponding to latencies of increased activation in the sensor-level analysis. Cortical areas showing significantly greater activation in response to words than pseudowords (in red/yellow) are highlighted and mean area activations plotted in the bar graphs; error bars show±1 s.e.m. adjusted to remove between-participant variance. Figure 2: Cortical sources underlying MEG sensor-level effects. Differences in minimum-norm source estimation of the brain responses elicited by words and pseudowords, averaged over all participants ( n =22). Images show mean source strength averaged across three windows corresponding to latencies of increased activation in the sensor-level analysis. Cortical areas showing significantly greater activation in response to words than pseudowords (in red/yellow) are highlighted and mean area activations plotted in the bar graphs; error bars show±1 s.e.m. adjusted to remove between-participant variance. Full size image Significantly stronger sources for words than for pseudowords were first observed in bilateral temporal lobes (left posterior temporal: t(21)=2.122, P =0.023; right temporal cortex: t(21)=3.021, P =0.0035) and simultaneously in the left lateral portion of the pre- and post-central cortex (t(21)=2.581, P =0.0085). In the second time window (110–170 ms), the lexicality effect reached significance exclusively in the right temporal cortex (t(21)=2.549, P =0.0095). Similar to the earliest effect observed, the late lexicality effect (320–520 ms) was supported by left posterior superior temporal cortex (t(21)=2.014, P =0.029) along with inferior frontal cortex (t(21)=1.993, P =0.0295), but was now underpinned by right anterior middle temporal activation as well (t(21)=1.762, P =0.047). As words and pseudowords presented in this study differed in terms of their lexical status, representing either familiar meaningful words or meaningless spoken analogues, the different brain responses between these stimuli appear to be best explained in terms of lexical processing in the brain. The most striking finding was the presence of an enhancement of brain responses to words compared with pseudowords, which started 50–80 ms after acoustic information allowed for unambiguous stimulus identification, suggesting extremely rapid lexical processing. Previous research on spoken word processing has typically reported neurophysiological effects indexing lexical processes in the N400 component, peaking at 350–400 ms after word onset, or starting within 200 ms at the earliest [17] , [18] , [19] . However, such onset-related early effects were observed when words were presented in phrasal context (not present here), and are attributable to the fact that the linguistic context ('he drinks his tea with milk and ...') led to anticipation of the critical items ('... sugar'), [27] , [28] , [29] , [30] therefore speeding the normal process of single word recognition. Moreover, to understand brain processes crucial for word recognition, which are absent for pseudowords, the relation between the onset of a word and a neurophysiological effect is not critical. At their respective onsets, both words and pseudowords activate the cohort of lexical representations in the brain that match the stimulus ('bi' may activate 'bill', 'bit', 'believe' and so on) [20] , [31] , [32] . Although there is evidence that the language system may engage in comprehension and semantic processing on the basis of incomplete lexical information, both at the behavioural [20] , [33] and the neurophysiological levels, [18] , [34] , [35] access to lexical representations of multiple candidates before lexical selection/word recognition point is thought to be partial and degraded, and to be reduced further when there are a high number of candidates [31] , as was the case in the present study. Only at the crucial point of word recognition (when 'bit' can be identified against the alternatives) can one specific word representation be accessed fully, whereas in the case of pseudowords, the word recognition process fails. To trace this important lexical effect neurophysiologically, it is therefore of utmost importance to measure brain responses not relative to word onset, but aligned to the point in time at which the acoustic information necessary for word recognition becomes available [21] . Thus, building upon existing psycholinguistic data and theory, in the present study we obtained word recognition points of our stimuli in a separate gating study. Although aligning responses to word recognition points was implemented in some previous studies, which showed a lexical enhancement of brain responses at 100–200 ms after the presentation of acoustic information required for word recognition, their results were based on mass repetition of few stimuli in the MMN paradigm, [21] , [22] which may have affected processing speed. In the present study, however, we define the neurophysiological lexicality effects relative to the word recognition points of a large sample of naturally spoken unique English words, each of which was presented only once in the experiment. The neurophysiological difference we observe may reflect the 'magic' moment in time when words are recognized, but pseudowords are not. We hasten to add that it is possible that other factors such as statistical properties of the initial consonant vowel (CV) syllables (for example, cohort frequency, which was controlled here to help define the recognition point, but not fully matched) may also contribute to the neurophysiological effects observed, and future research is therefore necessary to elucidate their potentially separable and specific contributions. The absence of a task directing listeners' attention to speech in the present experiment suggests that these earliest stages of lexical analysis may occur automatically, in the absence of focussed attention on linguistic input. The early lexical enhancement is largely supported by left perisylvian sources but also recruits sources in the right temporal lobe, indicating a bilateral contribution to the effect. The neurophysiological dissociation of words and pseudowords at 50–80 ms is the earliest marker of lexical processing of single words that has so far been reported in the literature. It may have been missed in previous studies for a number of reasons: first, stimuli may not have been fully matched or their physical features may have been too variable, leading to smearing of the short-lived early lexicality effects, which could be particularly problematic in studies that time-locked responses to word onsets rather than word recognition points; second, the inclusion of an active task may have interfered with the earliest automatic processing stage, and finally, in the case of MMN studies, repetition of the stimuli may have led to reduction of the earliest lexically sensitive response (repetition suppression). Following the earliest effect at 50–80 ms, we observed a lexical enhancement (110–170 ms) consistent with the previously reported enhancement of the MMN [21] . Our present data therefore suggest that the previously reported effect is distinct from and secondary to the earliest manifestation of lexical processing reported here. We also note that the timing of the second effect is similar to the earliest lexical manifestations reported from the visual domain, which occurred around 110–160 ms after the presentation onset of written words [14] , [16] . Although the sensor-level analysis suggested a predominant left-hemispheric involvement in this second effect, minimum-norm estimation (MNE) of the cortical sources indicated a role of the right anterior temporal lobe in its generation. This is in line with functional magnetic resonance imaging (fMRI) work implicating a role of this region in linguistic and conceptual processing [36] . The present data are in principle compatible with the possibility that lexical and semantic access emerge together during this time interval. There was also an effect in the N400 time window, the direction of which (lexical enhancement) is in contrast to the pseudoword enhancement observed in N400 studies where participants' attention is typically directed to the linguistic stimuli through the use of a task [37] , [38] . The inverted pattern we observe can be accounted for by the passive listening paradigm in which listeners were purposefully distracted from the auditory stimuli by a silent film. In line with the current data, elimination or even reversal of the N400 pseudoword enhancement has been seen previously in single-word EEG and MEG studies that also used a passive listening design [24] , [25] . In the same vein, a number of studies have suggested that the typically reported N400 effects reflect controlled processing of linguistic stimuli induced by the experimental tasks [39] , [40] , [41] , [42] . Although enhanced activation of the neural representations of words can occur automatically because of robustness of these neural circuits, in the absence of sufficient attentional resources no in-depth processing of pseudowords, which lack lexical representations, may occur. However, under appropriate task conditions where additional resources are available for the processing of pseudoword stimuli, there is intensified lexical search and possible re-analysis of the input when the initial attempt at mapping it to a single lexical entry fails. Such enhanced processing of pseudowords leads to an increase in the brain response magnitude, which often manifests as a pseudoword advantage in N400 studies, but is absent when attentional resources are diverted elsewhere, as we observe here. In addition to the evidence from electrophysiological investigations, this proposal received clear support and mechanistic explanation from neurobiologically based computational models of lexical representations and attention processes in the brain [43] . In sum, our findings demonstrate that the human brain is sensitive to differences between spoken words and pseudowords as early as 50 ms after the presentation of acoustic information required for word identification. Given that acoustic information at the cochlea reaches the primary auditory cortex within ∼ 15–20 ms, the current results suggest that the earliest cortical processes of word access and recognition may occur extremely rapidly after this point. Thus, our brain is capable of near-instantaneous access to information about spoken words, a capability that we suggest is important to the efficient and reliable use of language as our primary communication tool. Participants Twenty two right-handed (according to the Edinburgh inventory [44] ) native British English speakers (six male, mean age 24 years; range 18–35 years) with normal hearing and no record of neurological diseases took part in the study for financial compensation. Ethical approval was issued by Cambridge Psychology Research Ethics Committee (University of Cambridge) and informed written consent was obtained from all volunteers. Stimuli Stimuli were 108 distinct meaningful English words selected from a larger set within the MRC Psycholinguistic database that were monosyllabic, tri-phonemic, with a consonant-vowel-consonant (CVC) structure ending in [k], [t] or [p], and with a familiarity rating of >300 ( Supplementary Table S1 ). Importantly, the stimuli had a high cumulative CV cohort log frequency (mean of the summed log frequencies of all word forms in the cohort sharing the initial CV=34.1) based on monosyllabic words in the 17.9 million-token CELEX database [45] , driven by many lexical forms before the final consonant (mean CV cohort size=18). The cumulative CVC cohort log frequency was much lower (mean=4.9) and dominated by the word itself, indicating few competitors for the whole word form and ensuring successful word recognition only at the last phoneme. The words were accompanied by a set of 108 acoustically and phonological highly similar monosyllabic, tri-phonemic, CVC structure pseudowords that were matched with the words on mean log frequencies of their bigrams (words=5.2, pseudowords=5.1) and diphones (words=4.8, pseudowords=4.7). Pseudowords also had a high cumulative CV cohort log frequency (mean=24.6) and size (mean=13). Multiple tokens of the spoken stimuli uttered by a native female English speaker were recorded, and specific tokens were selected so that words and pseudowords were matched on durations before and after the plosion, and showed no differences in fundamental frequency (F0, the carrying frequency of the speech's acoustic signal) and total length. After this, all stimuli were normalized to have the same mean sound energy by matching the root mean square power of the acoustic signal ( Supplementary Fig. S1 ). In sum, stimuli were selected such that they could be uniquely identified as meaningful words or meaningless pseudowords only by a stimulus-final unvoiced plosive ([k], [t] or [p]) to ensure that the complete lexical information was available at the same time point for all stimuli. Word final unvoiced-stop consonants were chosen because of the minimal coarticulatory information available in the vowel period leading up to the plosion, and because the extended silent closure period preceding the final plosive provided an ideal prestimulus baseline that could be identical for words and pseudowords. To verify that the uniqueness point coincided with the onset of the plosion, a separate behavioural gating study [23] was carried out using all 216 stimuli by a group of 20 participants who did not take part in the MEG study. For each stimulus, 13 so-called 'gates' (that is, incomplete word fragments) were created: gate 1 comprised a fragment up to 200 ms before the offset of the vowel (mean 190 ms), gates 2–9 added increments of 10 ms up to the offset of the vowel, gate 10 corresponded to the onset of the plosion and gates 11–13 added a further three increments of 10 ms after the plosion. Stimuli were separated into two lists of 108 stimuli, each containing 18 words and pseudowords ending in [k], [t] and [p]. For each list, the fragments were presented binaurally in a random order such that stimuli and gate durations were mixed, to participants who had to report what they heard and their confidence in their response. The mean isolation point for the words, defined as the mean gate at which 80% of participants correctly identified the stimulus without subsequently changing their minds [46] , [47] occurred at gate 10, that is, at the plosion onset (s.e. ±1 ms). Mean confidence rating of at least 80% was not reached until gate 13. Procedure Participants ( n =22) were seated within a magnetically shielded room (IMEDCO GMBH, Switzerland). The sounds were presented binaurally at a comfortable hearing level through plastic tubing attached to foam earplugs, using the MEG-compatible sound-stimulation system (ER3A insert earphones, Etymotic Research, Inc., IL, USA). Stimuli were presented with a mean interstimulus offset-to-onset interval of 1500 ms (jittered in ±300 ms range) using E-Prime software (Psychology Software Tools, Inc., Pittsburgh, PA, USA). Participants were asked to ignore the auditory stimulation and focus their attention on watching a film (Wallace and Gromit); to ensure their compliance with the distracter task, they were warned that they would be tested on the film content. In a 5-option multiple-choice questionnaire conducted after the film (including one 'do not know' option), all participants performed above chance, indicating their compliance with the task. Participants also self-rated their attention to the film as higher than their attention to the sounds (t(21)=15.629, P <0.0001; for further details about these behavioural tests, see ref. 24 ). MEG recording and MRI data acquisition MEG was recorded continuously (sampling rate 1000 Hz, bandpass filter from 0.03 to 330 Hz) using a whole-head Vectorview system (Elekta Neuromag, Helsinki, Finland) containing 204 planar gradiometer and 102 magnetometer sensors. Head position relative to the sensor array was recorded continuously by using five head-position indicator (HPI) coils that emitted sinusoidal currents (293–321 Hz). Vertical and horizontal electro-oculograms were monitored with electrodes placed above and below the left eye and either side of the eyes. Before the recording, the positions of the HPI coils relative to three anatomical fiducials (nasion, left and right preauricular points) were digitally recorded using a 3-D digitizer (Fastrak Polhemus, Colchester, VA). Approximately 80 additional head points over the scalp were also digitized to allow the offline reconstruction of the head model and coregistration with individual MRI images. For each participant, high-resolution structural MRI images (T1-weighted) were obtained using a GRAPPA 3D MPRAGE sequence (TR=2250 ms; TE=2.99 ms; flip-angle=9° and acceleration factor=2) on a 3 T Tim Trio MR scanner (Siemens, Erlangen, Germany) with 1×1×1 mm isotropic voxels. MEG data processing To minimize the contribution of magnetic sources from outside the head and to reduce any within-sensor artifacts, the data from the 306 sensors were processed using the temporal extension of the signal-space separation technique [48] , implemented in MaxFilter 2.0.1 software (Elekta Neuromag); correlates of MEG signal originating from external sources were removed and compensation was made for within-block head movements (as measured by HPI coils). Subsequent processing was performed using the MNE Suite (version 2.6.0, Martinos Center for Biomedical Imaging, Charlestown, MA, USA) and the Matlab 6.5 programming environment (MathWorks, Natick, MA, USA). The continuous data were epoched relative to the onset of the stimulus-final plosion) between −50 and 800 ms, baseline-corrected over the prestimulus period of −50 to 0 ms and bandpass filtered between 1 and 30 Hz. Epochs were rejected when the magnetic field variation at any gradiometer or magnetometer exceeded 3,000 fT cm −1 or 6,500 fT, respectively, or when voltage variation at either bipolar electro-oculograms electrodes was >150 μV. For each participant, average event-related magnetic fields were computed for each condition (word and pseudoword), which resulted in a mean of 84 accepted trials in each condition. Overall signal strength of the event-related magnetic fields was quantified as the global SNR across all 306 sensors. To do this, we divided the amplitude at each time point by the s.d. in the baseline period for each sensor and then computed the square root of the sum of squares across all sensors. Time windows for analysis were selected on the basis of prominent peaks identified in the SNR collapsed across all conditions. Sensor-level analysis The event-related magnetic fields were quantified as the absolute amplitude of the 102 orthogonal gradiometer pairs by computing the square root of the sum of squares of the amplitudes of the two gradiometers in each pair. The resulting data were used to produce sensor-space grand averages across participants and for the subsequent statistical analysis on the sensor space data. For each time window, a t -test assessed whether mean global activation over the entire sensor array was larger for words compared with pseudowords, as predicted by previous research using auditory presentation of unattended words in a passive listening task (one-tailed). Follow-up analyses were performed on large clusters of the mean activations of 26 sensor pairs over the frontotemporal region at left and right hemispheres, where speech effects are typically maximal ( Supplementary Fig. S2 ). Source-level analysis Cortical sources of the observed neuromagnetic activity were estimated using signals from all 306 and the L2 MNE approach that models the recorded magnetic field distribution with the smallest amount of overall source activity [26] , [49] . Individual head models were created for each participant using segmentation algorithms (FreeSurfer 4.3 software, Martinos Center for Biomedical Imaging, Charlestown, MA, USA) to reconstruct the brain's cortical gray matter surface from structural MRI data. Further processing was performed using the MNE Suite 2.6.0 software. The original triangulated cortical surface was down-sampled to a grid by decimating the cortical surface with an average distance between vertices of 5 mm, which resulted in 10,242 vertices in each hemisphere. A single-layer boundary element model containing 5,120 triangles was created from the inner skull surface that was created using a watershed algorithm. Dipole sources were computed with a loose orientation constraint of 0.2 and no depth weighting, and with a regularization of the noise-covariance matrix of 0.1. Current estimates for individual participants were morphed to an average brain using five smoothing steps and, for visualisation, grand averaged over all 22 participants. Anatomically defined ROIs were created on the basis of the Desikan–Killiany Atlas parcellation of the cortical surface, [50] as implemented in the Freesurfer software package. We focused on activity in three main regions that are known to contribute to spoken language processing and, consistent with the previous research, produced the largest region-specific overall activity in the experiment ( Supplementary Fig. S3 ): superior, middle and inferior temporal (anterior and posterior segments), inferior frontal and pre- and post-central gyri (lateral segments). Regions in the superior, middle and inferior temporal gyri were sub-divided into anterior and posterior segments on the basis of parcellation of the cerebral cortex, as described by Rademacher and colleagues [51] where the anterior-posterior division corresponded approximately to the rostrolateral end of the first transverse sulcus; only the lateral segments of the pre- and post-central gyri were analysed. For the statistical analysis, mean amplitudes of the source currents were calculated over the time windows of interest defined in the sensor-level analysis, for the nine ROIs ( Supplementary Fig. S3 ). t -tests were performed for the selected regions in the left and right hemispheres to compare activation elicited by words and pseudowords. How to cite this article: MacGregor, L. J. et al . Ultra-rapid access to words in the brain. Nat. Commun. 3:711 doi: 10.1038/ncomms1715 (2012).